Interleukin-1α released from HSV-1-infected keratinocytes acts as a functional alarmin in the skin Herpes simplex virus-1 (HSV-1) is a human pathogen that utilizes several strategies to circumvent the host immune response. An immune evasion mechanism employed by HSV-1 is retention of interleukin-1β (IL-1β) in the intracellular space, which blocks the pro-inflammatory activity of IL-1β. Here we report that HSV-1-infected keratinocytes actively release the also pro-inflammatory IL-1α, preserving the ability of infected cells to signal danger to the surrounding tissue. The extracellular release of IL-1α is independent of inflammatory caspases. In vivo recruitment of leukocytes to early HSV-1 microinfection sites within the epidermis is dependent upon IL-1 signalling. Following cutaneous HSV-1 infection, mice unable to signal via extracellular IL-1α exhibit an increased mortality rate associated with viral dissemination. We conclude that IL-1α acts as an alarmin essential for leukocyte recruitment and protective immunity against HSV-1. This function may have evolved to counteract an immune evasion mechanism deployed by HSV-1. Pathogenic microorganisms have evolved to avoid detection by the host in which they proliferate. Their immune evasion strategies are essential for establishing infections; however, parallel to the pathogens acquiring mechanisms to avoid recognition by the host’s immune system, the host co-evolves to continue to sense and eliminate microorganisms. Herpes simplex virus-1 (HSV-1) is a human pathogen that establishes primary and secondary infections of skin and mucosal epithelial cells, and latency in sensory nerve ganglia [1] . HSV-1 achieves productive local infection of mammalian cells by inhibiting both inflammatory and apoptotic pathways. The virus can spread to the brain or internal organs such as the liver and lungs; however, such cases are rare as the host normally develops strong and effective immune protection against dissemination of the virus [1] , [2] . Complications from HSV-1 infections are typically only observed in immune-compromised individuals and neonates in whom the immune system is still developing [3] , [4] , [5] . However, when either encephalitis or disseminated disease occur, the morbidity and mortality rates are high. Interleukin-1 (IL-1) represents two pleiotropic cytokines, IL-1α and IL-1β, essential for both innate and adaptive immune responses [6] . IL-1α is expressed in high levels in keratinocytes, whereas myeloid cells such as macrophages are a major source of IL-1β. Interestingly, while both IL-1α and IL-1β signal through the extracellular domain of the transmembrane IL-1 receptor type 1 (IL-1R1), both cytokines are initially synthesized as intracellular pro-proteins. The pro-IL-1α and pro-IL-1β can be cleaved by the cysteine proteases calpain and caspase-1, respectively [6] . Processing of pro-IL-1β to the mature IL-1β is required for functional activity and extracellular release of the cytokine [6] . In contrast, pro-IL-1α is functionally active and may be released from dying cells [6] . As such, it is believed to act as an alarmin; a protein stimulating recruitment of inflammatory cells to sites of tissue damage after the protein is released from the dying cells [7] . It has been shown that necrotic cells release IL-1α in vitro and that these cells can recruit neutrophils when administered in vivo [8] , [9] . However, an alarmin function of IL-1α during a natural physiological response involving in vivo -induced cell death has not been reported previously. Caspase-1, which cleaves pro-IL-1β, is activated following assembly of inflammasomes, multimeric protein complexes activated by microorganisms and tissue damage [10] . Caspase-4 and caspase-5 (mouse homologue: caspase-11) are functionally related to caspase-1, as they also initiate inflammation [10] . Interestingly, while many activators of the inflammasomes, including pathogens, lead to cleavage and secretion of IL-1β, HSV-1-infected cells fail to release IL-1β [11] , [12] , despite inflammasome assembly and caspase-1 activation [12] , [13] , [14] . In fibroblasts, at least, this appears to be because of degradation of IFI16 initiated by the immediate early HSV-1 protein ICP0 and retention of caspase-1 within actin fibres [12] . Hence, HSV-1 appears to elude IL-1β-dependent immune responses by preventing secretion of IL-1β. The mechanisms whereby IL-1α is released from cells are less well understood and whether HSV-1 targets these as an immune-evasion strategy is unknown. Despite extensive studies of HSV-1’s immune-evasion strategies in fibroblasts and myeloid cells, less is known about how the virus is sensed in epithelial cells in the skin and mucosal membranes where it causes tissue damage and blisters through cytopathic effects. We demonstrate here that skin keratinocytes release IL-1α following HSV-1 infection in an inflammatory caspase-independent manner. This release is important for recruitment of leukocytes to the epidermis during the very early stages of skin infection. Furthermore, IL-1R1-deficient mice are more susceptible to dissemination of the virus and the resulting lethal outcomes. Hence, IL-1α acts as an alarmin signalling danger in response to HSV-1 infection. This mechanism may have evolved to counter the IL-1β targeting HSV-1 immune-evasion strategy. HSV-1-infected keratinocytes release IL-1α HSV-1 evades the inflammatory functions of IL-1β by preventing secretion of the mature cytokine [11] , [12] . If a similar immunosuppressive strategy is in place to neutralize the related function of IL-1α is unknown. Since keratinocytes express ~10-fold more IL-1α than IL-1β [15] , [16] , [17] and are one of the major cell types in which HSV-1 replicates, we were interested in the role of these cells in signalling danger to the host. Using direct and indirect approaches, it has previously been demonstrated that keratinocytes release IL-1α following infection with the HSV-1 isolates KOS and F [18] , [19] . TLR3 plays an important role in protecting the central nervous system from HSV-1 infections, presumably through detection of double-stranded RNA that may be produced during the viral life cycle [20] , [21] . We previously reported that poly(I:C), a synthetic double-stranded RNA analogue, induced chemokine expression in keratinocytes and that this induction is partially dependent upon IL-1α release from the cells [22] . As predicted, based on these observations, we found elevated levels of IL-1α in medium from cells treated with poly(I:C) ( Fig. 1a ). Similar levels of IL-1α were present in the medium from HSV-1 NS isolate-infected human ( Fig. 1a ) and mouse ( Supplementary Fig. 1 ) primary keratinocytes 6 and 24 h post infection (human Fig. 1a ; 24-h mouse Supplementary Fig. 1 ). While increased IL-1β levels were detected after poly(I:C) treatment, analogous changes in IL-1β levels were not detected after HSV-1 infection ( Fig. 1b ). The IL-1β released by keratinocytes in response to poly(I:C) has previously been shown to be the inactive pro-IL-1β form [23] . Hence, our data demonstrate that IL-1α, but not IL-1β, is successfully released from keratinocytes infected with the HSV-1 NS isolate. 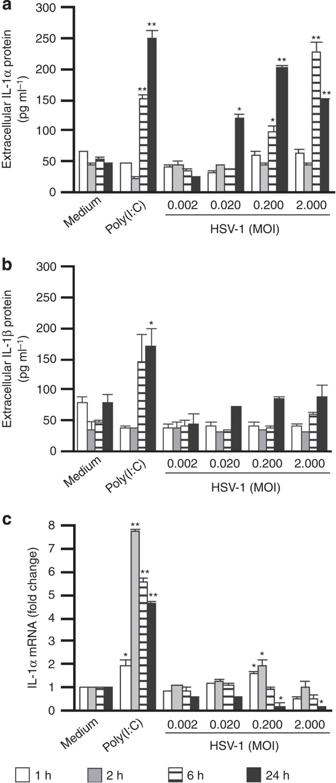Figure 1: HSV-1-infected keratinocytes release IL-1α. Primary human keratinocytes were treated with medium only, 25 μg ml−1poly(I:C) or HSV-1 as indicated. After 1 h, cells were rinsed with PBS and fresh medium without agents was added. Cultures were allowed to incubate further for 1 (white bars), 2 (grey), 6 (striped) or 24 (black) h before conditioned medium (a,b) and cells (c) were collected. (a,b) Extracellular levels of IL-1α (a) and IL-1β (b) proteins (in the culture medium) were determined with ELISA. (c) IL-1α mRNA levels were determined using the ΔΔCtmethod with GAPDH as the internal reference gene and medium-only treated cells as the external reference point. Data points (n=2) are means±s.d. from one representative experiment of at least three independent experiments with similar outcomes. *P<0.05 (compared with medium only,t-test); **P<0.01. Figure 1: HSV-1-infected keratinocytes release IL-1α. Primary human keratinocytes were treated with medium only, 25 μg ml −1 poly(I:C) or HSV-1 as indicated. After 1 h, cells were rinsed with PBS and fresh medium without agents was added. Cultures were allowed to incubate further for 1 (white bars), 2 (grey), 6 (striped) or 24 (black) h before conditioned medium ( a , b ) and cells ( c ) were collected. ( a , b ) Extracellular levels of IL-1α ( a ) and IL-1β ( b ) proteins (in the culture medium) were determined with ELISA. ( c ) IL-1α mRNA levels were determined using the ΔΔ C t method with GAPDH as the internal reference gene and medium-only treated cells as the external reference point. Data points ( n =2) are means±s.d. from one representative experiment of at least three independent experiments with similar outcomes. * P <0.05 (compared with medium only, t -test); ** P <0.01. Full size image Released IL-1α is derived from a pre-formed pool of protein In agreement with a previous report examining IL-1α mRNA expression in mouse keratinocytes infected with the HSV-1 KOS isolate [19] , we found that levels of the IL-1α mRNA were significantly downregulated 24 h post infection with the HSV-1 NS isolate ( Fig. 1c ). The absence of an increase in IL-1α mRNA expression correlating with the levels of IL-1α protein detected in the medium ( Fig. 1a ) suggests that the released IL-1α is primarily derived from a pre-formed pool of protein. Analyses of cellular IL-1α further supported this interpretation, as levels of IL-1α decreased in a time- and viral titre (multiplicity of infection (MOI))-dependent manner ( Fig. 2a ). Significantly higher levels of intracellular than extracellular IL-1α (compare Fig. 2a to Fig. 1a ) were detected. This likely reflects autocrine functionality of IL-1α leading to internalization and degradation of the cytokine following receptor engagement [24] , [25] , [26] , [27] , [28] , [29] . In summary, our data ( Figs 1 and 2 ) show that pre-formed cellular IL-1α is released into the extracellular milieu in response to HSV-1 infection. 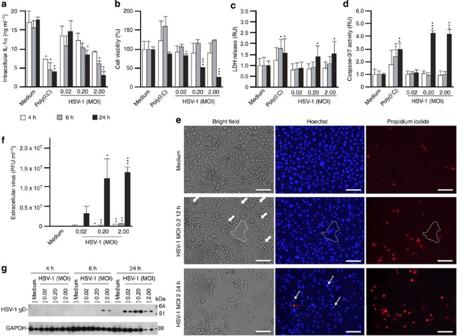Figure 2: IL-1α release precedes cell death and correlates with HSV-1 replication. Mouse (a–d,f,g) and human (e) keratinocytes were treated with poly(I:C) or were infected with HSV-1 as described inFig. 1and indicated in each panel. (a) Cellular levels of IL-1α and GAPDH were determined with ELISA. Cellular IL-1α levels are shown standardized against levels of GAPDH. (b) Viability of cells was determined by measuring intracellular levels of ATP. (c) Loss of membrane potential was measured via levels of lactate dehydrogenase (LDH) in the culture medium. (d) Activity of the apoptosis executioner caspases-3/7 was determined enzymatically. (b–d) Cell viability/death readouts were standardized against medium-only-treated cells at the equivalent time point. (e) HSV-1 cytopathic effects were detected using bright-field and fluorescence microscopy and nuclear staining with Hoechst and propidium iodide. A giant multinucleated cell containing four nuclei is outlined. Additional giant multinucleated cells containing >2 nuclei are indicated with white block arrows. Horizontal red line arrow indicates a cell with full Hoechst stain brightness surrounded by cells with reduced brightness. White line arrows indicate cells at different stages of nuclear condensation associated with apoptosis. Representative images from two independent experiments are shown. Scale bars=200 μm. (f) Numbers of virus particles in the cell culture medium were determined using quantitative PCR. (g) Equal volumes of cellular protein extracts were examined with Western blot analysis. The HSV-1 protein gD was detected using serum from HSV-1-infected mice. Levels of host cell proteins were indicated by detection of GAPDH (rabbit anti-GAPDH, FL-335). Two independent samples per time point and treatment are shown. Full images of western blots are shown inSupplementary Fig. 2. (a–d,f) Data points (n=2) are means±s.d. from one representative experiment of at least three independent experiments with similar outcomes. *P<0.05 (compared with medium only,t-test); **P<0.01; ***P<0.001. Figure 2: IL-1α release precedes cell death and correlates with HSV-1 replication. Mouse ( a – d , f , g ) and human ( e ) keratinocytes were treated with poly(I:C) or were infected with HSV-1 as described in Fig. 1 and indicated in each panel. ( a ) Cellular levels of IL-1α and GAPDH were determined with ELISA. Cellular IL-1α levels are shown standardized against levels of GAPDH. ( b ) Viability of cells was determined by measuring intracellular levels of ATP. ( c ) Loss of membrane potential was measured via levels of lactate dehydrogenase (LDH) in the culture medium. ( d ) Activity of the apoptosis executioner caspases-3/7 was determined enzymatically. ( b – d ) Cell viability/death readouts were standardized against medium-only-treated cells at the equivalent time point. ( e ) HSV-1 cytopathic effects were detected using bright-field and fluorescence microscopy and nuclear staining with Hoechst and propidium iodide. A giant multinucleated cell containing four nuclei is outlined. Additional giant multinucleated cells containing >2 nuclei are indicated with white block arrows. Horizontal red line arrow indicates a cell with full Hoechst stain brightness surrounded by cells with reduced brightness. White line arrows indicate cells at different stages of nuclear condensation associated with apoptosis. Representative images from two independent experiments are shown. Scale bars=200 μm. ( f ) Numbers of virus particles in the cell culture medium were determined using quantitative PCR. ( g ) Equal volumes of cellular protein extracts were examined with Western blot analysis. The HSV-1 protein gD was detected using serum from HSV-1-infected mice. Levels of host cell proteins were indicated by detection of GAPDH (rabbit anti-GAPDH, FL-335). Two independent samples per time point and treatment are shown. Full images of western blots are shown in Supplementary Fig. 2 . ( a – d , f ) Data points ( n =2) are means±s.d. from one representative experiment of at least three independent experiments with similar outcomes. * P <0.05 (compared with medium only, t -test); ** P <0.01; *** P <0.001. Full size image Extracellular release of IL-1α precedes cell death execution HSV-1 is well known to be cytopathic to epithelial cells, including keratinocytes. We found that viability of HSV-1-infected keratinocytes was significantly reduced after 24 h ( Fig. 2b ). This loss of viability correlated with loss of membrane potential ( Fig. 2c ) and activation of the apoptosis executioner caspases-3/7 ( Fig. 2d ). Formation of multinucleated giant cells could be detected after 12 h at MOI<1 ( Fig. 2e , MOI 0.2, block arrows). At the 24-h time point, most HSV-1-infected cells exhibited clear signs of cytopathic effects. However, it is noteworthy that most cells still maintained membrane potential as indicated by the exclusion of propidium iodide ( Fig. 2e ). Decreased brightness of the Hoechst stain, an indication of apoptosis initiation ( Fig. 2e , red arrow indicates a cell with full brightness), could also be detected in many HSV-1-infected cells ( Fig. 2e ). Interestingly, the apparent mixed cell death events were detected only at time points past that at which the first IL-1α was released from the cells ( Figs 1a and 2a ). This shows that the release of IL-1α is an active process preceding execution of cell death programmes. Release of IL-1α correlates with viral replication The observation that IL-1α is released from cells earlier ( Figs 1a and 2a ) than the cells die ( Fig. 2b–e ) prompted us to examine the timing of viral replication in our model system. Viral particles could be detected in culture medium from infected cells as early as 4 h post infection and levels increased over time ( Fig. 2f ). In agreement with this, trace levels of the HSV-1 glycoprotein D (gD) could be detected in cells at the 4-h time point, when cells were infected with the highest viral titre used ( Fig. 2g and Supplementary Fig. 2 ). Higher levels of HSV-1 gD were observed at later time points where gD could also be detected in cells infected with lower HSV-1 titres ( Fig. 2g and Supplementary Fig. 2 ). At the 24-h time point, the levels of HSV-1 gD correlated with the MOI, except for the highest titre used (MOI=2.0). The observed lower levels of HSV-1 gD at the latter data point correlated with decreased levels of host cell glyceraldehyde 3-phosphate dehydrogenase (GAPDH) and is consistent with the reduced viability of cells ( Fig. 2b ) and initiation of cell death ( Fig. 2c,d ). The timing of viral protein ( Fig. 2g and Supplementary Fig. 2 ) and particle ( Fig. 2f ) production correlated with the release of IL-1α ( Figs 1a and 2a ). Hence, our observations suggest that the release of IL-1α is initiated by events associated with replication of HSV-1 in the host cell. HSV-1 activates inflammatory caspases in keratinocytes It has been reported that the inflammasome is activated in response to HSV-1 infection in fibroblasts in vitro and in the eye in vivo [13] , [14] . However, keratinocytes have not been examined previously. Analyses of the human inflammatory caspases revealed that one or more of these were significantly activated 6 h post infection ( Fig. 3 ). Similar observations were made using mouse keratinocytes ( Supplementary Fig. 3 ). Therefore, our data document that HSV-1 does activate inflammasomes in keratinocytes. 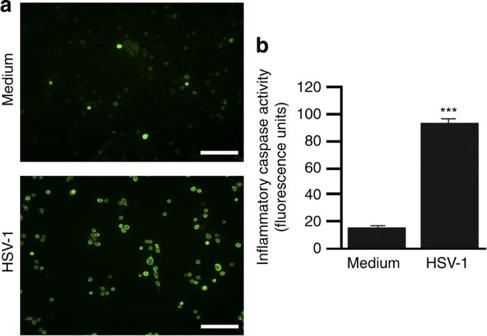Figure 3: Inflammatory caspases are activated in HSV-1-infected keratinocytes. Human keratinocytes were treated with vehicle or HSV-1. After 6 h, cells were incubated for 2 h with a fluorescent probe for the active site of the inflammatory caspases 1, 4 and 5. Unbound probe was removed by washing the cells with fresh medium and activated inflammatory caspases visualized using a fluorescence microscope (a, representative images shown, scale bars=200 μm) or quantified using a plate reader (b, means±s.d.). ***P<0.001 (compared with medium only,t-test). One representative experiment of three independent experiments is shown. Figure 3: Inflammatory caspases are activated in HSV-1-infected keratinocytes. Human keratinocytes were treated with vehicle or HSV-1. After 6 h, cells were incubated for 2 h with a fluorescent probe for the active site of the inflammatory caspases 1, 4 and 5. Unbound probe was removed by washing the cells with fresh medium and activated inflammatory caspases visualized using a fluorescence microscope ( a , representative images shown, scale bars=200 μm) or quantified using a plate reader ( b , means±s.d.). *** P <0.001 (compared with medium only, t -test). One representative experiment of three independent experiments is shown. Full size image IL-1α can be released independently of inflammatory caspases HSV-1 is believed to activate innate immune mechanisms via double-stranded RNA generated during the viral life cycle and poly(I:C) has been widely used to simulate these responses (for example, refs 30 , 31 ). Inflammatory caspases have been linked to poly(I:C)-induced release of pro-IL-1β [23] and IL-36γ [15] . Since both poly(I:C) and HSV-1 trigger the release of IL-1α ( Fig. 1 ), we hypothesized that these responses were also dependent upon inflammatory caspases. As predicted, we found that poly(I:C)-induced release of IL-1α could be blocked by a caspase inhibitor specific to the inflammatory caspases ( Fig. 4a ). Surprisingly, IL-1α levels in the medium from HSV-1-infected wild-type cells and cells deficient of both caspase-1 and caspase-11, the inflammatory caspases in mice, were not significantly different (Fig. 4b ). This demonstrates that HSV-1-induced IL-1α is independent of the inflammatory caspases and further suggests that HSV-1 and poly(I:C) activate innate immune mechanisms in keratinocytes through, at least in part, different pathways. 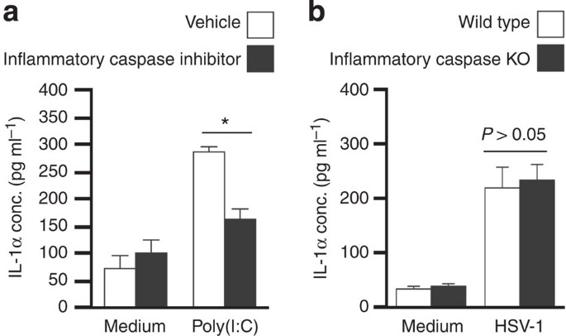Figure 4: Poly(I:C)-, but not HSV-1, stimulated IL-1α release is inflammatory caspase-dependent. (a) Human primary keratinocytes were pre-treated with vehicle (white bars) or an inflammatory caspase-specific inhibitor (black bars) for 30 min before addition of medium or 25 μg ml−1poly(I:C). Culture medium was collected after 12 h and IL-1α levels determined using ELISA. (b) Mouse primary keratinocytes isolated from wild-type (white bars) and inflammatory caspase-deficient (black bars) mice were infected with HSV-1 (0.2 MOI) as described inFig. 1. Control cells were treated with medium only. IL-1α released into the culture medium 24 h post infection was quantified using a mouse IL-1α-specific ELISA. (a,b) Data points (n=3) represent means±s.d. Each experiment was repeated at least twice with similar outcomes. *P<0.05 (compared with medium only,t-test). Figure 4: Poly(I:C)-, but not HSV-1, stimulated IL-1α release is inflammatory caspase-dependent. ( a ) Human primary keratinocytes were pre-treated with vehicle (white bars) or an inflammatory caspase-specific inhibitor (black bars) for 30 min before addition of medium or 25 μg ml −1 poly(I:C). Culture medium was collected after 12 h and IL-1α levels determined using ELISA. ( b ) Mouse primary keratinocytes isolated from wild-type (white bars) and inflammatory caspase-deficient (black bars) mice were infected with HSV-1 (0.2 MOI) as described in Fig. 1 . Control cells were treated with medium only. IL-1α released into the culture medium 24 h post infection was quantified using a mouse IL-1α-specific ELISA. ( a , b ) Data points ( n =3) represent means±s.d. Each experiment was repeated at least twice with similar outcomes. * P <0.05 (compared with medium only, t -test). Full size image IL-1 does not affect primary and secondary infections To explore the physiological role of HSV-1-induced IL-1α release from skin keratinocytes, we employed the flank model of HSV-1 infection. Briefly, in this model mice are scratch-inoculated with HSV-1 on the skin (primary infection site). From here, the virus spreads first through retrograde nerve migration to the dorsal root ganglion, and subsequently through anterograde migration back into the skin, where it causes secondary skin disease along the affected nerves. At the virus dose utilized here, death may occur from days 10 to 14 post infection because of viral dissemination to vital organs such as the brain, liver and lungs. Death is sometimes preceded by weight loss ( Supplementary Fig. 4 ). Infected wild-type and IL-1R1 KO mice revealed no strain-specific differences in viral titres at the primary infection sites 2 days post- infection ( Supplementary Fig. 5 ). This demonstrates that wild-type and the IL-1R1 KO mice are equally susceptible to the primary HSV-1 infection. Secondary lesions along the sensory nerves started to appear on day 5 in both wild-type and IL-1R1 KO mice (see below). Total areas of lesions were comparable in wild-type and IL-1R1 KO mice ( Supplementary Fig. 6 ). Hence, HSV-1 appears to spread through the nerves of wild-type and IL-1R1 KO mice at a similar rate. Inflammation is indistinguishable in the processed skin IL-1 has pleiotropic effects upon the immune system [6] . Therefore, we examined markers of immunological activation in full thickness skin, comprising both dermis and epidermis, from primary and secondary lesions ( Fig. 5 ). IL-1α can activate T cells, including γδ T cells, and hence modulate IL-17A expression [32] . Surprisingly, there were no statistically significant differences between the wild-type and the IL-1R1 KO mice in terms of TCR δ chain (an indirect measure of γδ T-cell numbers) and IL-17A mRNA expression ( Fig. 5a ). 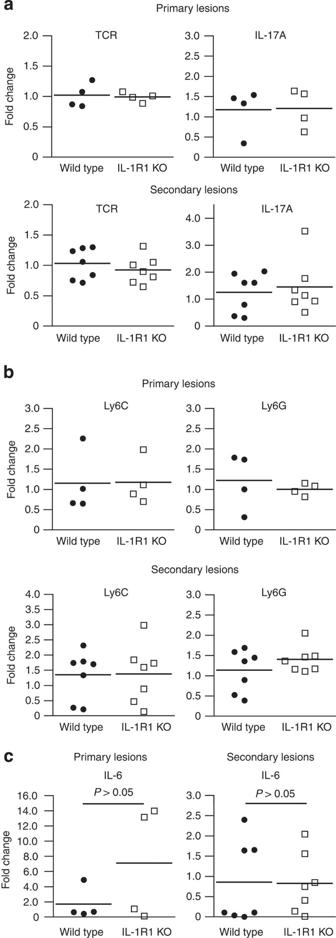Figure 5: Skin inflammation appears independent of IL-1R1 in processed full thickness skin. Wild-type (black circles) and IL-1R1 KO (white boxes) mice (n=4–7 per group) were infected with 1.5 × 106PFU HSV-1 on flank skin. Five days post infection, the primary and secondary skin lesions were collected separately and expression of cell type marker (TCR δ chain (a), Ly6C and Ly6G (b)) and cytokine (IL-17A (a) and IL-6 (c)) mRNAs examined with real-time RT-PCR. The mRNA levels were standardized against GAPDH and expressed as fold change as described inFig. 1. No statistically significant (t-test) differences between wild-type and IL-1R1 KO mice were identified. Figure 5: Skin inflammation appears independent of IL-1R1 in processed full thickness skin. Wild-type (black circles) and IL-1R1 KO (white boxes) mice ( n =4–7 per group) were infected with 1.5 × 10 6 PFU HSV-1 on flank skin. Five days post infection, the primary and secondary skin lesions were collected separately and expression of cell type marker (TCR δ chain ( a ), Ly6C and Ly6G ( b )) and cytokine (IL-17A ( a ) and IL-6 ( c )) mRNAs examined with real-time RT-PCR. The mRNA levels were standardized against GAPDH and expressed as fold change as described in Fig. 1 . No statistically significant ( t -test) differences between wild-type and IL-1R1 KO mice were identified. Full size image Neutrophils and monocytes/macrophages are among the cell types initially recruited to sites of sterile inflammation [33] . IL-1α is known to have neutrophil and monocyte targeting pro-inflammatory activity [22] , [32] , [34] , [35] ; hence, we examined recruitment of these cell types into HSV-1-infected skin of wild-type and IL-1R1 KO mice using the granulocyte markers Ly6C and Ly6G. In addition, we were surprised to find no statistically significant differences between wild-type and IL-1R1 KO mice ( Fig. 5b ). We further examined expression of the pro-inflammatory cytokine IL-6. While levels of the IL-6 mRNA were found to vary dramatically from mouse to mouse, we observed no statistically significant differences in IL-6 expression between wild-type and IL-1R1 KO mice ( Fig. 5c ). While these expression analyses are only indirect indications of leukocyte recruitment into the skin, they suggest that overall skin inflammation was indistinguishable in wild-type and IL-1R1 KO mice. IL-1 signalling promotes spatial recruitment of leukocytes The outcome of the expression analyses ( Fig. 5 ) prompted us to examine the three-dimensional localization of inflammation within lesions ( Fig. 6 ). As mentioned earlier, we did not find that external appearances of lesions progressed differently in wild-type and IL-1R1 KO mice ( Fig. 6 , photographs). Microscopically, however, differences between wild-type and IL-1R1 KO mice were identified. Primary lesions exhibited extensive leukocyte recruitment into the skin and the epidermis was absent ( Fig. 6a ). Interestingly, while in wild-type mice a dense infiltrate could be detected where the epidermis previously was, this inflammation appeared more diffuse in IL-1R1 KO mice ( Fig. 6a ). 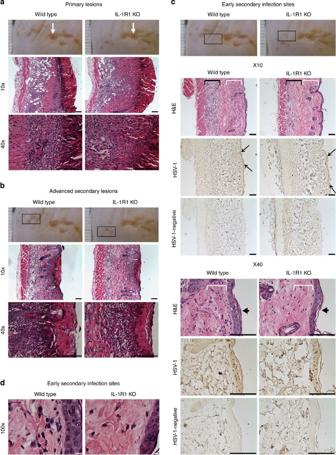Figure 6: IL-1R1 controls spatial leukocyte recruitment to the epidermis. Wild-type and IL-1R1 KO mice were scratch-inoculated with 1.5 × 106PFU HSV-1. Five days post infection, primary infection sites (a, white arrows), advanced secondary lesions (b, boxes) and early secondary infection sites (c,d, boxes) were collected, fixed and examined with haematoxylin–eosin staining. (c) Consecutive tissue sections were additionally stained with HSV-1 antiserum (HSV-1) or secondary antibody only (HSV-1 negative). (c) White and black brackets indicate positions of subepidermal and -cutaneous leukocyte infiltration, respectively. Black line arrows demarcate borders of early secondary infection sites. Black block arrows indicate centres of early secondary infection sites. Representative images from one of the two experiments are shown (n=3–5 per group per experiment). Black scale bars=100 μm. White scale bar=10 μm. Figure 6: IL-1R1 controls spatial leukocyte recruitment to the epidermis. Wild-type and IL-1R1 KO mice were scratch-inoculated with 1.5 × 10 6 PFU HSV-1. Five days post infection, primary infection sites ( a , white arrows), advanced secondary lesions ( b , boxes) and early secondary infection sites ( c , d , boxes) were collected, fixed and examined with haematoxylin–eosin staining. ( c ) Consecutive tissue sections were additionally stained with HSV-1 antiserum (HSV-1) or secondary antibody only (HSV-1 negative). ( c ) White and black brackets indicate positions of subepidermal and -cutaneous leukocyte infiltration, respectively. Black line arrows demarcate borders of early secondary infection sites. Black block arrows indicate centres of early secondary infection sites. Representative images from one of the two experiments are shown ( n =3–5 per group per experiment). Black scale bars=100 μm. White scale bar=10 μm. Full size image To avoid confounding by the potential effects of viral scratch inoculation and secondary leukocyte recruitment, we further examined inflammation in and around sites of secondary lesions ( Fig. 6b , boxes) and early secondary infection sites ( Fig. 6c,d , boxes). The latter were yet to develop into lesions, that is, the epidermis was intact. Interestingly, sites of early epidermal HSV-1 infection, where the virus had not yet destroyed the cells ( Fig. 6c , black line arrows), contained high numbers of leukocytes just below the epidermis in wild-type mice ( Fig. 6c , white brackets; magnified in Fig. 6d ). On the basis of morphology, these cells appeared to be primarily neutrophils and macrophages ( Fig. 6d ). These cell populations were greatly reduced in IL-1R1 KO mice ( Fig. 6c,d , white brackets). It is noteworthy that the timing of leukocyte recruitment in vivo to infected sites, before destruction of the epidermis ( Fig. 6c,d ), correlates with the release of IL-1α from infected keratinocytes before detectable cell death ( Figs 1 and 2 ). Hence, in vivo release of IL-1α from HSV-1-infected cells appears to play an essential role in spatial recruitment of leukocytes to sites immediately adjacent to the HSV-1 infection; in particular, the very early stages of infection before and/or during cell death and tissue damage. IL-1R1 provides protection against lethal outcomes HSV-1 infections can lead to serious complications with a potential fatal outcome [3] , [4] , [5] . Therefore, we examined the prospective mortality rates of wild-type and IL-1R1 KO mice following flank HSV-1 infection. Approximately 25% of the wild-type mice died from the infection during a 16-day period ( Fig. 7a ). The median survival time of the IL-1R1 KO mice was only 13 days ( Fig. 7a ) and approximately only 40% of the mice were alive on day 16. This represents a statistically significant reduction in survival of the IL-1R1 KO mice compared with wild-type mice and demonstrates that IL-1R1 signalling plays an important role in protecting the host against HSV-1 infections. 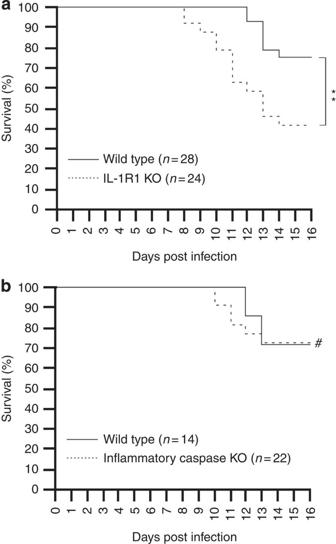Figure 7: IL-1R1, but not inflammatory caspases, provides protection from lethal outcome. Wild-type (black lines,a,b), IL-1R1 KO (dotted line,a) and inflammatory caspase KO (dotted line,b) mice were infected with 1.5 × 106PFU HSV-1 on the flank and survival monitored for 16 days. Data shown are pooled fromFigs 4aand3bindependent experiments.nindicates the total number of mice per strain used. **P<0.01; #P>0.05 (Mantel–Cox and Gehan–Breslow–Wilcoxon tests). Figure 7: IL-1R1, but not inflammatory caspases, provides protection from lethal outcome. Wild-type (black lines, a , b ), IL-1R1 KO (dotted line, a ) and inflammatory caspase KO (dotted line, b ) mice were infected with 1.5 × 10 6 PFU HSV-1 on the flank and survival monitored for 16 days. Data shown are pooled from Figs 4a and 3b independent experiments. n indicates the total number of mice per strain used. ** P <0.01; # P >0.05 (Mantel–Cox and Gehan–Breslow–Wilcoxon tests). Full size image Both IL-1α and IL-1β can signal via IL-1R1. While IL-1α is active in its pro-form, IL-1β requires processing (for example, by caspase-1) for functional activity and can be released from pyroptotic cells in a caspase-11-dependent manner [6] , [36] . Mice deficient of the inflammatory caspases, caspase-1 and caspase-11, exhibited the same survival rate as wild-type mice ( Fig. 7b ). Consequently, a role for inflammatory caspase-dependent IL-1β in IL-1R1-mediated protection ( Fig. 7a ) can be excluded. Hence, our data suggest that the protection conferred by IL-1R1 is because of IL-1α engagement. Wild-type and IL-1R1 KO mice show similar disease symptoms It has previously been reported that TLR3-deficient mice have an increased HSV-2 infectivity of astrocytes [21] . The same study indicated that the TLR3 KO mice developed constipation, bladder retention and paralysis following vaginal infection with HSV-2 (ref. 21 ). In our flank model, HSV-1-infected mice developed a severe bowel dysfunction syndrome without any bias towards either strain ( Supplementary Fig. 7 ). We did not find bladder retention to be associated with HSV-1 infection ( Supplementary Fig. 7 ) nor did we observe paralysis. Weight differences of wild-type and IL-1R1 KO survivors at the end of the experiment (day 16, Fig. 8a ) were not statistically significant. The wild-type and IL-1R1 KO moribund mice, although their average weight was lower than that of survivors, also had similar weights ( Fig. 8a ). Furthermore, serum IL-6 levels were comparable in moribund wild-type and IL-1R1 KO mice ( Supplementary Fig. 8 ). Hence, IL-1R1 KO mice appear to develop disease similar to that of wild-type mice. 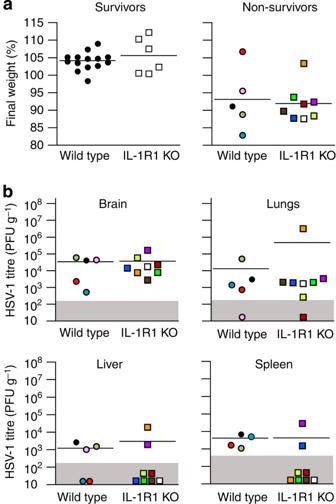Figure 8: Wild-type and IL-1R1 KO mice exhibit similar biodistribution of HSV-1. Wild-type (circles,n=19) and IL-1R1 KO (squares,n=14) mice were infected with 1.5 × 106PFU HSV-1 and weight and behaviour monitored for up to 16 days. Moribund mice were identified based on a dramatic and abnormal decrease in activity and were killed before collection of tissues. (a) Weight at the end of the experiment (day of killing for moribund mice and day 16 for survivors) is represented as the percentage of weight at the beginning of the experiment. (b) HSV-1 viral loads were determined using quantitative PCR in moribund mice. Grey boxes indicate the limit of detection. Each colour represents a single mouse. Data shown are pooled from two independent experiments. No statistically significant (t-test) differences between wild-type and IL-1R1 KO mice were identified. Figure 8: Wild-type and IL-1R1 KO mice exhibit similar biodistribution of HSV-1. Wild-type (circles, n =19) and IL-1R1 KO (squares, n =14) mice were infected with 1.5 × 10 6 PFU HSV-1 and weight and behaviour monitored for up to 16 days. Moribund mice were identified based on a dramatic and abnormal decrease in activity and were killed before collection of tissues. ( a ) Weight at the end of the experiment (day of killing for moribund mice and day 16 for survivors) is represented as the percentage of weight at the beginning of the experiment. ( b ) HSV-1 viral loads were determined using quantitative PCR in moribund mice. Grey boxes indicate the limit of detection. Each colour represents a single mouse. Data shown are pooled from two independent experiments. No statistically significant ( t -test) differences between wild-type and IL-1R1 KO mice were identified. Full size image IL-1R1 deficiency increases viral dissemination To better understand the nature of the increased mortality of the IL-1R1 KO mice, viral loads in organs from moribund mice were determined. Somewhat expected, given the neurotropic behaviour of the HSV-1 NS strain, HSV-1 could be detected in the brains of moribund mice ( Fig. 8b ). However, we did not observe a statistically significant difference in brain viral burden between wild-type and IL-1R1 KO mice ( Fig. 8b ). In humans, HSV can cause disseminated disease involving internal organs such as the lungs and liver [3] , [4] , [5] . It also has been reported that different strains of HSV can proliferate in the spleens of infected mice [37] . Here we detected HSV-1 in the lungs, liver and spleen of moribund wild-type and IL-1R1 KO mice ( Fig. 8b ). Interestingly, no trends towards statistically significant differences in viral titres between wild-type and IL-1R1 KO mice were detected ( Fig. 8b ). Since wild-type and IL-1R1 KO mice exhibit similar biodistribution of HSV-1 following flank infection ( Fig. 8b ), our data demonstrate that IL-1R1 does not regulate susceptibility to infection in target organs per se . Instead, the protective function of IL-1R1 ( Fig. 7a ) appears to be mediated by limiting viral dissemination from the skin or nerves to other organs, that is, more IL-1R1 KO than wild-type mice succumb to fatal disease ( Figs 7a and 8 ). IL-1α is believed to be an alarmin as the protein is released from dying cells and has pro-inflammatory properties [7] , [9] ; however, direct documentation of this function in vivo has been elusive. Our data demonstrate that the cytopathic HSV-1 triggers extracellular release of IL-1α, but not IL-1β, by keratinocytes from a pre-formed pool of the cytokine ( Figs 1 and 2 ). During in vivo HSV-1 infection, IL-1R1 signalling is required for recruitment of leukocytes to sites immediately adjacent to infected cells in the epidermis ( Fig. 6 ), a tell-tale sign of alarmin activity [7] . Hence, our study demonstrates, for the first time, the function of IL-1α as an alarmin during viral skin infections. Only microorganisms that avoid detection by the host’s immune response succeed as pathogens. HSV-1 has developed several immune evasion strategies, one of which involves blocking the function of caspase-1 and extracellular release of the pro-inflammatory mature IL-1β [11] , [12] . The ability of HSV-1-infected keratinocytes to release the alarmin IL-1α preserves the capacity of the infected cells to communicate the present danger and may represent an evolutionary adaptation of the host to counter viral immune-evasion strategies. Such co-evolution of the host may explain why most HSV-1 infections are self-limiting and typically only immune-deficient individuals are at risk of developing serious complications such as disseminated disease and encephalitis [3] , [4] , [5] . Cells can die through many different pathways and mechanisms. As of 2012, there were at least 12 biochemically distinct types of cell death [38] . HSV-1 is cytopathic to keratinocytes; however, the process of cell death remains unclear. It has been reported that HSV-1 initiates apoptosis in the early stages of cell infection [31] , [39] , [40] , [41] , [42] , [43] . However, as the viral cycle progresses, the virus expresses proteins involved in blocking the execution of apoptosis [31] , [39] , [40] , [41] , [42] , [43] . The latter is believed to be an immune-evasion mechanism [31] , [39] , and the initiated cell death may in fact be part of the host’s response aimed at eliminating the infection [31] , [39] , [40] , [41] , [42] , [43] . Similarly, autophagy and necroptosis may be initiated and inhibited by HSV-1 (refs 31 , 44 ). We previously reported that poly(I:C), a double-stranded RNA analogue often utilized to mimic viral infections [30] , [31] , activates pyroptosis in keratinocytes [15] . Pyroptosis is an inflammatory form of programmed cell death dependent upon the inflammatory caspases. We here found that poly(I:C)-triggered IL-1α release was inflammatory caspase-dependent ( Fig. 4a ). Surprisingly, extracellular IL-1α accumulation induced by HSV-1 was independent of the inflammatory caspases ( Fig. 4b ). This could suggest that the initiating events are different, for example, poly(I:C) engages TLR3 (ref. 23 ), whereas HSV-1 activates IFI16 (ref. 45 ). Alternatively, the activating event leading to extracellular release of IL-1α is the same and the differential requirement for inflammatory caspases is because of the ability of HSV-1 to modulate the inflammasome pathway [11] , [12] leading to divergence of the pathways. Cellular release of IL-1α correlated with viral replication ( Fig. 2f,g ) and IL-1α appeared in cell culture medium before detectable signs of cell death ( Figs 1 and 2 ). However, while the release of IL-1α appears to precede cell lysis, it may still be linked to cell death as an early, programmed, step of self-destruction. Further studies will be required to elucidate how keratinocytes die and release IL-1α following infection with HSV-1. Recruitment of immune cells to sites of infection is a pre-requisite for initiation of adaptive immunity. We found that IL-1α·IL-1R1 signalling promotes leukocyte placement next to HSV-1-positive cells in the skin ( Fig. 6 ). In addition, IL-1R1 is crucial for preventing lethal systemic disease ( Figs 7a and 8 ), indicating a role in regulating protective immunity. IL-1R1 is the receptor for both IL-1α and IL-1β. IL-1β must be proteolytically processed, for example, by caspase-1 (ref. 6 ), and undergo unconventional protein secretion in a frequently caspase-11-dependent manner [36] . Ablation of caspase-1 and caspase-11 did not affect survival of mice in our experimental system ( Fig. 7b ). This excludes caspase-1/caspase-11-dependent IL-1β release from contributing to the observed IL-1R1-protective function ( Fig. 7a ). However, alternative pathways, for example, caspase-8 (ref. 46 ) and cathepsin C [47] , for IL-1β activation have been discovered in recent years. Yet, HSV-1-infected fibroblasts and macrophages fail to release processed IL-1β because of a poorly understood mechanism deployed by the virus [11] , [12] . In addition, we observed that keratinocytes do not secrete IL-1β in response to HSV-1 ( Fig. 1b ). Hence, IL-1β release from HSV-1-infected cells appears unlikely as a contributing factor in our infection model. It remains a possibility that caspase-1/caspase-11-independent release of IL-1β from non-HSV-1-infected cells, for example, in response to tissue damage caused by the virus, could contribute to the here-reported IL-1R1-dependent survival ( Fig. 7a ). A definitive conclusion regarding the possible role of IL-1β in this system will require the use of IL-1α and IL-1β KO mice. Such studies may also reveal the specific mechanism(s) of IL-1R1-dependent protective immunity against HSV-1. Evolutionary development of multiple pathways for IL-1β activation may represent host counter measures for viral immune-evasion strategies. Inhibition of IL-1 signalling via transgenic overexpression of the IL-1 receptor antagonist, IL-1Ra, has been shown to protect against ocular damage caused by HSV-1 strain RE infection [48] . This protective effect was mediated via a reduction in neutrophil recruitment and angiogenesis [48] . In HSV-1 strain NS-infected skin we observed a dramatic influx of neutrophils in advanced lesions ( Fig. 6 ), and it is very likely that the recruited neutrophils contributed to the tissue damage leading to skin lesions ( Fig. 6 ). However, we did not detect differences in lesion development and progression between wild-type and IL-1R1 KO mice ( Fig. 6 and Supplementary Fig. 6 ). As discussed above, the immune system has several levels of apparent redundancies built into it to counter immune-evasion mechanisms developed by pathogens. Since the eye is an immune-privileged site, there may be less redundancy in the pro-inflammatory mechanisms here compared with non-privileged sites such as the skin. Consequently, a tissue-protective effect of inhibiting IL-1·IL-1R1 signalling may be more readily detected in an immune-privileged site, for example, the eye, with fewer pro-inflammatory pathways. Here our reported data demonstrate that keratinocytes are capable of signalling danger to the surrounding tissue via IL-1α ( Fig. 1 ). This alarm signal is essential for recruitment of leukocytes to sites of infection ( Fig. 6 ) and development of protective immunity ( Fig. 7 ). Future studies exploring how IL-1α is released from infected cells and how this cytokine supports immune functions may lead to novel immune-enhancement strategies for immunocompromised patients with, or at risk of, disseminated disease and/or encephalitis. Cell cultures and protein extracts Primary human neonatal keratinocytes (Life Technologies) were maintained in EpiLife Medium supplemented with EpiLife Defined Growth Supplement and gentamicin (25 μg ml −1 , Life Technologies). Alternatively, the cells were maintained in Defined Keratinocyte Serum-Free Medium (Life Technologies). Mouse primary keratinocytes were isolated from newborn pups (24–72 h). The epidermis and dermis were separated after incubation with 0.25% trypsin at 37 °C for 45 min or over night at 4 °C. Epidermal sheets were minced and nutated at 4 °C for 45 min in culture medium. Cells were plated on rat-tail type I collagen-coated (4.3 μg cm −1 , BD Bioscience) plates and maintained in Keratinocyte Serum-Free Medium (Life Technologies) supplemented with mouse epidermal growth factor (10 ng ml −1 , Sigma-Aldrich), calcium chloride (45 μM, final concentration), bovine pituitary extract (140 μg ml −1 , Life Technologies) and gentamicin. African green monkey kidney epithelial cells (Vero, generously provided by Dr Harvey M. Friedman, University of Pennsylvania, Philadelphia, PA, USA) were maintained in DMEM (Life Technologies) supplemented with 50 mM HEPES, 2 mM glutamine, 5% fetal bovine serum and 10 μg ml −1 gentamicin. Cellular protein extracts were prepared by freeze-thawing cells three times in M-PER Mammalian Protein Extraction Reagent (Thermo Scientific) supplemented with 1% Mammalian Cells Protease Inhibitor Cocktail (Sigma-Aldrich) and 10 mM EDTA. Production of virus and infections The clinical HSV-1 isolate NS (kindly provided by Dr Harvey M. Friedman) was produced in Vero cells. Viral titres were determined with plaque assays. Briefly, 10-fold serial dilutions were prepared on ice in the DMEM serum-free medium. Vero cells were grown in a 12-well plate and washed with PBS with calcium and magnesium immediately before infection. Subsequently, cells were incubated with 200 μl virus from the serial dilutions at 37 °C for 1 h. After incubation, the cells were washed and overlayed with 1 ml per well of a 1:1 mixture of twofold medium (DMEM low-glucose powder (Sigma) with supplements) and 1.2% low melting temperature agarose. Plaques were counted ~48 h post infection. For experimental infections, cells were incubated with viral MOI as indicated for 1 h in serum/protein-free medium. Cells were rinsed with PBS before addition of virus-free complete culture medium. Cells and conditioned medium were collected at the indicated time points. Detection and imaging of cell death and viability Lactate dehydrogenase in cell culture medium was measured using the Cytotoxicity Detection Kit (Roche) according to the manufacturer’s instructions. Caspase-3/7 activity and cell viability (intracellular ATP) was monitored using the Caspase-Glo 3/7 and CellTiter-Glo, respectively, luciferase assay systems (Promega) following the manufacturer’s instructions. For imaging, cells were cultured on glass bottom dishes (MatTek) coated with rat-tail collagen type I (BD Biosciences). Nuclei were sequentially stained with Hoechst 33342 and propidium iodide (ImmunoChemistry Technologies). Inflammatory caspase activity and inhibition Activation of the human inflammatory caspases, caspase-1, -4 and -5 (mouse homologues caspase-1 and -11) was monitored using FAM-YVAD-FMK according to the manufacturer’s (ImmunoChemistry Technologies) instructions. Inflammatory caspases were inhibited with Caspase-1 Inhibitor VI (EMD Biosciences). The inhibitor was solubilized in dimethylsulfoxide (vehicle control) and added to cultures 30 min before stimulation with medium only or poly(I:C) (Sigma-Aldrich). Final concentration of the inhibitor was 20–50 μM. Expression analyses Levels of human and mouse IL-1α, IL-1β and IL-6 protein were determined using appropriate species-specific enzyme-linked immunosorbent assays (ELISAs) according to the manufacturers’ (R&D Systems and Peprotech) instructions. GAPDH protein levels were determined using a direct ELISA approach as previously described [15] . Briefly, cell lysates were coated on 96-well plates and GAPDH detected by sequential incubation with rabbit anti-GAPDH (FL-335, 6 pg ml −1 ; Santa Cruz Biotechnology), goat anti-rabbit IgG-HRP (250 ng ml −1 , Santa Cruz Biotechnology) and ABTS chromogen (Thermo Scientific). RNA was isolated from cell cultures using RNeasy (Qiagen) according to the manufacturer’s instructions. Skin was homogenized in QIAzol using a Bio-Gen PRO200 homogenizer equipped with interchangeable Multi-Gen 7XL probes (PRO Scientific) and RNA isolated using RNeasy Plus Universal kit (Qiagen) according to the manufacturer’s instructions. Relative gene expression was determined with real-time PCR using the comparative ΔΔ C t method and GAPDH as the internal reference/housekeeping gene. RNA (1 μg per sample) was reverse-transcribed at 37 °C for 1.5 h using 1 μg oligo(dN) 6 , 5.5 U RNAguard Ribonuclease Inhibitor (GE Healthcare) and 10 U AMV reverse transcriptase (Promega) according to the manufacturer’s instructions. Inactivation of AMV was performed at 95 °C for 10 min The following primers were used for analyses of gene expression in human cells: hIL-1α-forward, 5′-CAGTGAAATTTGACATGGGTG-3′; hIL-1α-reverse, 5′-CAGGCATCTCCTTCAGCAG-3′; hGAPDH-forward, 5′-GGTCGGAGTCAACGGATTTG-3′; hGAPDH-reverse, 5′-TGGGTGGAATCATATTGGAAC-3′. For analyses of gene expression in mouse skin, the following primers were used: mIL-1α-forward, 5′-TGAGTCGGCAAAGAAATCAAG-3′; mIL-1α-reverse, 5′-AGTGAGCCATAGCTTGCATC-3′; mTCR delta-forward, 5′-GGAGACTACGGTTCCTGAAAG-3′; mTCR delta-reverse, 5′-AAATGTGGTGGTGAAGGGT-3′; mIL-17A-forward, 5′-TTTTCAGCAAGGAATGTGGA-3′; mIL-17A-reverse, 5′-TTCATTGTGGAGGGCAGA-3′; mIL-6-forward, 5′-GATGGATGCTACCAAACTGG-3′; mIL-6-reverse, 5′-TCTGAAGGACTCTGGCTTTG-3′; mLy6c1-forward, 5′-GGATGGACACTTCTCACACTAC-3′; mLy6c1-reverse, 5′-GCAGTCCCTGAGCTCTTTC-3′; mLy6G-forward, 5′-GCACATGAAAGAGGCAGTATTC-3′; mLy6G-reverse, 5′-GAGACATTGAACAGCACACATAG-3′; mGAPDH-forward, 5′-CTTGTGCAGTGCCAGCC-3′; mGAPDH-reverse, 5′-GCCCAATACGGCCAAATCC-3′. Equal volumes of cellular protein extracts were separated using SDS–PAGE and transferred to polyvinylidene difluoride membranes. The membranes were blocked with 5% milk-protein and HSV-1 proteins detected using serum (1/100 dilution) from mice infected with HSV-1. GAPDH (detected with FL-335, 67 ng ml −1 ) was used as the loading control. In vivo HSV-1 infections C57BL/6, IL-1 receptor type 1 (IL-1R1) KO and caspase-1/11 (inflammatory caspases) KO mice were obtained from Jackson Laboratory and bred in house under specific pathogen-free conditions. Both KO strains were on the C57BL/6 genetic background. The Temple University Institutional Animal Care and Use Committee approved all animal procedures. Male and female mice of ages 7–12 weeks were used. Mice were matched for age and sex in each individual experiment. Mice were denuded the day before infections. Mice were scratch-inoculated with 1.5 × 10 6 PFU HSV-1 on the right flank. Development of secondary lesions along the sensory nerves was photo-documented and lesion sizes determined using ImageJ. Blood was collected by cardiac puncture immediately after killing. Titration of HSV-1 in tissue Primary infection sites were collected using 8-mm biopsy punches. Each lesion was divided into two and one half used for DNA isolation. Organs were frozen and crushed into a powder with autoclaved mortar and pestle over dry ice. DNA was extracted from skin and organs using the DNeasy Blood & Tissue kit from Qiagen according to the manufacturer’s instructions. Viral titres at the primary infection sites and organs were determined using equal amounts of total DNA and quantitative real-time PCR with the primer/probe set 5′-CGACCAACTACCCCGAT-3′ (forward primer), 5′-CACTATGACGACAAACAAAATCAC-3′ (reverse primer) and VIC-CAGTTATCCTTAAGGTCTC-MGBNFQ (probe). PCR amplification was performed using the TaqMan Gene Expression Master Mix (Applied Biosystems) on an Eppendorf Realplex [2] Mastercycler for primary infection site analysis and an Applied Biosystems StepOnePlus Real-Time PCR System for organ tissue analysis. Histology and immunohistochemistry Mouse skin was fixed in 4% formaldehyde, buffered in PBS and processed for standard haematoxylin–eosin staining at the Histotechnology Facility (Wistar Institute). For immunohistochemistry, paraffin sections were deparaffinized in xylene and passed through decreasing concentrations of alcohol. Sections were microwaved in 10 mM Sodium Citrate (pH 6.0) and then allowed to cool to room temperature. Slides were treated with 3% hydrogen peroxide followed by blocking with 5% goat serum, 20% egg whites and biotin solution (Vector). HSV-1 was detected using serum collected 8 days post-HSV-1 infection of wild-type mice. Serum was added as primary antibody and incubated at room temperature for 1 h. ECL anti-mouse IgG, horseradish peroxidise-linked whole antibody (GE Healthcare) was used as secondary antibody (1/100 in PBS) and allowed to incubate for 30 min at room temperature. Bound antibodies were visualized with DAB Plus substrate and chromogen (Ultravision Plus Detection System, Thermo Scientific). Slides were mounted with Shandon-Mount (Thermo Scientific). Image acquisition Images were acquired using an Olympus BX60 microscope equipped with Olympus × 10/0.25 and × 240/0.65 lenses and fluorescence capability. Digital acquisition was achieved using the SPOT Insight camera (2 mega sample) and software (version 4.5) from Diagnostic Instruments. Imaging processes were Mac operated at room temperature. Statistical analyses Statistical significance was determined using t , Mantel–Cox and Gehan–Breslow–Wilcoxon tests. Data are shown as arithmetic means±s.d. unless specified otherwise. All experiments were performed at least three times with similar outcomes. How to cite this article: Milora, K. A. et al. Interleukin-1α released from HSV-1-infected keratinocytes acts as a functional alarmin in the skin. Nat. Commun. 5:5230 doi: 10.1038/ncomms6230 (2014).